Probing electric field control of magnetism using ferromagnetic resonance Exchange coupled CoFe/BiFeO 3 thin-film heterostructures show great promise for power-efficient electric field-induced 180° magnetization switching. However, the coupling mechanism and precise qualification of the exchange coupling in CoFe/BiFeO 3 heterostructures have been elusive. Here we show direct evidence for electric field control of the magnetic state in exchange coupled CoFe/BiFeO 3 through electric field-dependent ferromagnetic resonance spectroscopy and nanoscale spatially resolved magnetic imaging. Scanning electron microscopy with polarization analysis images reveal the coupling of the magnetization in the CoFe layer to the canted moment in the BiFeO 3 layer. Electric field-dependent ferromagnetic resonance measurements quantify the exchange coupling strength and reveal that the CoFe magnetization is directly and reversibly modulated by the applied electric field through a ~180° switching of the canted moment in BiFeO 3 . This constitutes an important step towards robust repeatable and non-volatile voltage-induced 180° magnetization switching in thin-film multiferroic heterostructures and tunable RF/microwave devices. Much recent research has been devoted to realizing fast, compact and low-power magnetoelectric random access memories (MERAM) [1] , [2] , [3] , [4] based on electric field (E-field) control of magnetization. Multiferroic materials with simultaneous ferroelectricity and magnetism provide a pathway to achieving strong magnetoelectric coupling with efficient voltage control of magnetism, and compact and power-efficient electric field-tunable magnetic devices [1] , [2] , [3] , [4] . A variety of ‘magnetoelectric-multiferroics’ such as magnetic/ferroelectric [5] , [6] , [7] , [8] , [9] , [10] , [11] , [12] and magnetic/multiferroic [13] , [14] , [15] , [16] , [17] heterostructures have been investigated, which are providing pathways to novel electric field-tunable radio frequency (RF)/microwave signal processing devices [5] , magnetic field sensors [6] , MERAM devices [7] and voltage-tunable magnetoresistance devices [8] . Several magnetoelectric coupling mechanisms have been explored to achieve efficient electric field control of magnetism, for example, strain-mediated magnetoelectric coupling [9] , [10] , [11] , [12] , [18] , [19] , spin-polarized charge-mediated magnetoelectric coupling [20] , [21] , [22] , [23] , [24] , [25] and voltage control of carrier-mediated magnetism in dilute magnetic semiconductors [26] , [27] , [28] . Strain-mediated magnetoelectric coupling in thin-film magnetic/ferroelectric heterostructures on substrates can be diminished due to substrate clamping effects [6] , [18] , [19] , while spin-polarized charge-mediated magnetoelectric coupling can only be observed in ultra-thin (<1 nm) magnetic thin films [20] , [21] , [22] , [23] , [24] , [25] , which puts a limit on its application in real magnetoelectric devices. Finally, voltage control of carrier-mediated magnetism in dilute magnetic semiconductors has been challenging at room temperature [26] , [28] . The room temperature single-phase multiferroic, BiFeO 3 (BFO), has attracted a lot of recent research interest due to the coexistence of robust ferroelectricity ( P ) and antiferromagnetism ( L ) [13] , [14] , [15] , [16] , [17] , [29] , [30] , [31] , [32] , [33] , [34] , [35] , [36] and a weak canted magnetic moment ( M C ). In bulk BFO, the weak moment results from the canting of the magnetic sublattices due to the Dzyaloshinskii–Moriya interaction [14] as predicted by the density functional theory [14] and confirmed experimentally [30] , [36] . E-field control of magnetism, magnetoresistance [13] , magnetic anisotropy [15] and magnetization [16] in a ferromagnetic layer exchange coupled to BFO layer has been most recently reported. Nevertheless, one fundamental question has remained open: does the canted moment in this system reverse direction on the application of an electric field? In a recent paper, we used a combination of ab initio computation, magnetotransport measurements and photoemission electron microscopy studies to demonstrate that the canted moment can indeed switch by 180° when the ferroelectric polarization is switched by 180°, particularly in a (001)-oriented epitaxial film that is comprised of a periodic ferroelectric domain pattern [37] . To emphasize and validate the results of these studies, we have carried out a very detailed electric field-dependent ferromagnetic resonance (FMR) study of exactly the same heterostructure (CoFe/BFO). The FMR results directly validate, confirm and quantify the electric field-dependent magnetotransport results. Phase field-based theoretical studies present complementary validation of the experimental results and are consistent with the ab initio theoretical results. FMR of the CoFe layer is used to probe both the coupling between the CoFe and BFO and the electric field modulation of this coupling. We find that an out-of-plane (OOP) electric field on BFO induces an anisotropic in-plane (IP) change in the CoFe layer FMR field, which is 8±1 mT along the magnetic easy axis of the CoFe layer and ≈0 mT along the magnetic hard axis. The switching of the FMR field, which occurred at the same voltage as the switching of the BFO ferroelectric polarization, is repeatable over at least 100 reversals. This robust and repeatable switching in the CoFe/BFO heterostructure provides a potential mechanism for compact and power-efficient MERAM and voltage tunable RF microwave devices. We provide a model for the modulation of the FMR field as a consequence of the α ≈180° switching of the canted moment of the BFO layer that is exchange coupled to the CoFe layer. Further, we extracted the effective coupling field (~5.7±0.4 mT) and canted moment switching angle (178°±11°) quantitatively by FMR measurements. Voltage tunable magnetic film/BFO heterostructures enable next generation of compact, fast, energy-efficient and voltage-controllable MERAM devices. Moreover, in this work, the tunability of CoFe at X-band RF/microwave frequency also provides the opportunity to realize voltage tunable RF/microwave devices, such as, filters, phase shifters and antennas, which are widely used in aircraft, satellite, radar and mobile communication systems. Preparation and imaging of CoFe/BFO Ferromagnetic-multiferroic thin-film heterostructures of Pt (2.5 nm)/Co 0.9 Fe 0.1 (2.5 nm)/BiFeO 3 (200 nm)/SrRuO 3 (SRO; 10 nm) were grown onto (110)-oriented DyScO 3 (DSO) substrates with a SRO layer as the bottom electrode using pulsed laser deposition [33] . The resulting epitaxial BFO layer exhibits a characteristic, two-domain structure consisting of a one-dimensional, quasi-periodic array of 71° domains [31] ; we use this as a model system to probe the coupling to the ferromagnetic CoFe. The Pt (2.5 nm)/Co 0.9 Fe 0.1 (2.5 nm) bilayers were deposited on BFO films under a 20-mT in situ bias magnetic field along the DSO (1–10) direction, leading to a well-defined IP magnetic easy axis in the CoFe layer. The ferroelectric domain structure of the BFO layer was imaged by measuring the intensity of the back-scattered electrons as shown in Fig. 1a [17] . We image the magnetic structure of the CoFe layer at zero magnetic field using scanning electron microscopy with polarization analysis (SEMPA) [38] . By measuring the spin polarization of secondary electrons, SEMPA directly measures the local vector magnetization in the CoFe layer [39] . An example of an IP magnetization image is shown in Fig. 1b . Comparison of the SEMPA and back-scattered electron images clearly shows the close correlation between the magnetic structure of the CoFe film and the quasi-periodic, striped ferroelectric domain structure of the underlying BFO layer. Within a stripe, which is about 250 nm wide, the magnetization is aligned or antialigned with the IP surface projection of the electric polarization which is along BFO <111> directions [13] . We note that this alignment with the projection of the polarization is fortuitous; indeed, on this surface, the canted moment also projects parallel to the polarization and the moment in the CoFe layer couples to this. Furthermore, the magnetization switches by ~90° between adjacent stripes with the net or average magnetization perpendicular to the stripes as is illustrated in the magnified image in Fig. 1c . The deviation from perfect 90° switching of the magnetization between adjacent stripes is due to the competition between intra-layer exchange coupling within the CoFe film and coupling to the BFO. Micromagnetic modelling of this structure, Supplementary Fig. 1 and Fig. 2 , confirms this interpretation and yields an effective interfacial coupling field of ~7 mT (ref. 17 ). The striped structure forms two types of magnetic domains in this as-prepared remnant state: one with the net magnetization parallel to the net IP polarization direction (yellow/red striped region in Fig. 1c ) and the other with net IP magnetization antiparallel (blue/cyan striped region). The coexistence of parallel and antiparallel magnetization orientations, along with other measurements, demonstrates that the magnetic coupling to the BFO leads to a net uniaxial rather than unidirectional anisotropy in the CoFe layer [17] . 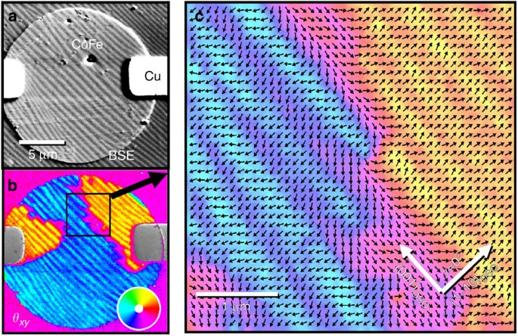Figure 1: Ferroelectric domain structure of BFO and ferromagnetic domain structure of CoFe with polarization analysis. (a) The ferroelectric domain structure imaged using the back-scattered electron (BSE) intensity with a CoFe thin-film circular disk and Cu electrode on the side. (b) The simultaneously acquired SEMPA image of the magnetic structure. The magnetization direction,θxy, is represented by colour as indicated by the colour wheel. (c) An enlarged view of the magnetization with arrows added to show the measured magnetization directions and the relationship to the DSO substrate. Figure 1: Ferroelectric domain structure of BFO and ferromagnetic domain structure of CoFe with polarization analysis. ( a ) The ferroelectric domain structure imaged using the back-scattered electron (BSE) intensity with a CoFe thin-film circular disk and Cu electrode on the side. ( b ) The simultaneously acquired SEMPA image of the magnetic structure. The magnetization direction, θ xy , is represented by colour as indicated by the colour wheel. ( c ) An enlarged view of the magnetization with arrows added to show the measured magnetization directions and the relationship to the DSO substrate. 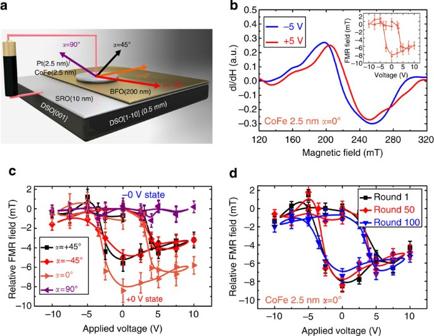Figure 2: FMR measurements of CoFe/BFO multiferroic heterostructure. (a) Schematic of CoFe (2.5 nm)/BFO (200 nm) multiferroic heterostructure for FMR measurements at varying anglesαbetween the magnetic field and the easy axis; (b) FMR spectra of CoFe/BFO multiferroic heterostructure measured at open circuit after applying +5 V and −5 V atα=0°.Upper right inset is the relative FMR field dependence on applied voltage; (c) relative FMR field dependence after applied voltage pulses along different orientations of the magnetic field; (d) relative FMR field versus applied voltage pulses after 50 and 100 cycles of a 10-V sinusoidal voltage. Error bars inb–dare defined as the s.d. of five FMR measurements for each FMR data. Full size image Figure 2: FMR measurements of CoFe/BFO multiferroic heterostructure. ( a ) Schematic of CoFe (2.5 nm)/BFO (200 nm) multiferroic heterostructure for FMR measurements at varying angles α between the magnetic field and the easy axis; ( b ) FMR spectra of CoFe/BFO multiferroic heterostructure measured at open circuit after applying +5 V and −5 V at α =0°.Upper right inset is the relative FMR field dependence on applied voltage; ( c ) relative FMR field dependence after applied voltage pulses along different orientations of the magnetic field; ( d ) relative FMR field versus applied voltage pulses after 50 and 100 cycles of a 10-V sinusoidal voltage. Error bars in b – d are defined as the s.d. of five FMR measurements for each FMR data. Full size image FMR measurements of CoFe/BFO Field-dependent FMR at X-band (9.5 GHz) under different applied voltages (across the BFO layer) was measured as schematically shown in Fig. 2a , with α being the angle between the applied magnetic field direction and the net magnetic easy axis of CoFe layer. The sample was rotated from 0° to 360° in the FMR measurement system. Voltage pulses (100 ms) with varying amplitudes from 10 to −10 V were applied across the BFO layer and all the FMR spectra at open circuit after each voltage pulse were recorded at a fixed α . As shown in Fig. 2b at α =0°, we observe a large voltage-induced FMR field shift (the difference between blue and red curve at zero crossing) of 8±1 mT after applying +5 V (red) and −5 V (blue) voltage pulse amplitudes. By tracing the FMR field (that is, the zero crossing of the magnetic field of the FMR spectrum in Fig. 2b ) after applying different voltage pulses, we obtain the dependence of the FMR field on the voltage pulse amplitude. The upper right inset of Fig. 2b shows a typical square, hysteretic dependence on voltage. Figure 2c shows the FMR field dependence on the applied voltage pulses along different magnetic field orientations, α =−45°, 0°, 45° and 90°, from the CoFe layer magnetic easy axis. The largest voltage-induced FMR field change is 8±1 mT at α =0°, that is, when the magnetic field was applied along the easy axis. At α =−45° or 45°, we observe a relatively smaller FMR field shift with the maximum FMR shift being 5±1 mT. The hysteretic FMR field dependence on voltage pulse amplitude means that it is switched back and forth by voltage pulses between two states, identified as the +0 V state and −0 V state; in Fig. 2c . However, there is no obvious hysteretic behaviour at α =90°, and the maximum FMR shift is comparable to the measurement noise level (≈0.5 mT). To test the repeatability of the voltage control of the FMR field shift, we then apply a sinewave voltage signal with an amplitude of 10 V (frequency=0.167 Hz ) across the thickness direction of the BFO layer. We measure the dependence of the FMR field on applied voltage pulse after switching the voltage 50 and 100 times by the sinewave as shown in Fig. 2d . Similar hysteresis loops of the FMR field shift at α =0° are observed after 50 and 100 ferroelectric switching cycles indicating a robust, non-volatile and repeatable voltage-induced FMR field shift. 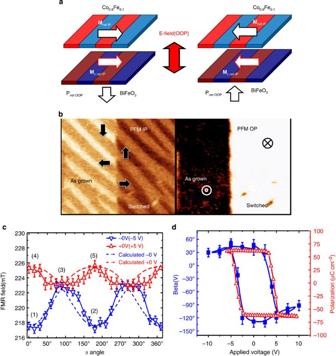Figure 3: Study and analysis of voltage impulse-induced polarization and canted moment switches in CoFe/BFO. (a) Schematic of coupling between magnetic momentMof CoFe layer coupled and the IP component ofMCin BFO layer, whereMCcan be tuned by an OOPEfield. (b) The IP (left) and OOP (right) PFM images with arrows indicating the polarization orientation in each stripe before (left half of each image) and after applying an OOPEfield. (c) Angular dependence of the FMR field after applying different voltage pulses, +5 V (red) and −5 V (blue), at each angleα. Dash line represents theoretical simulation results. (d) Dependence ofβ, the angle between the IP projection of the canted moment in the red BFO domain and the easy axis, on applied voltage pulse, compared with the polarization of the BFO layer versus applied voltage measured at 9.5 GHz. Error bars incare defined as the s.d. of five FMR measurements for each FMR data. Error bars indare deducted by the error of FMR measurements. Figure 3a represents the schematic of CoFe/BFO bilayer two-domain stripe-like structure, in which the magnetization of CoFe can be tuned by an OOP E-field. While Fig. 3b shows the corresponding IP (left) and OOP (right) piezo force microscopy (PFM) images with polarization orientations manipulated by an OOP E-field. Figure 3c shows the angular dependence of the magnetic coupling and illustrates the main result of our measurements. After the +5-V pulse was applied across the BFO layer, the FMR field dependence on α was switched from the blue curve (−0 V state) to the red one (+0 V state) at a fixed α angle, corresponding to the +0-V state of FMR field. A subsequent −5 V voltage pulse switched the angular dependence of the FMR field back to the blue curve (−0 V state). The angular dependence of the blue curve indicates that the CoFe magnetization is parallel to the effective magnetic coupling field from BFO near 0° and 180°. On the other hand, the angular dependence of the red curve shows that by changing the electric polarization, the CoFe magnetization, which has not changed due to the large magnetic field applied for the FMR measurements, now lies in a direction that is antiparallel to the effective magnetic coupling field from BFO, leading to a higher FMR field. Figure 3: Study and analysis of voltage impulse-induced polarization and canted moment switches in CoFe/BFO. ( a ) Schematic of coupling between magnetic moment M of CoFe layer coupled and the IP component of M C in BFO layer, where M C can be tuned by an OOP E field. ( b ) The IP (left) and OOP (right) PFM images with arrows indicating the polarization orientation in each stripe before (left half of each image) and after applying an OOP E field. ( c ) Angular dependence of the FMR field after applying different voltage pulses, +5 V (red) and −5 V (blue), at each angle α . Dash line represents theoretical simulation results. ( d ) Dependence of β , the angle between the IP projection of the canted moment in the red BFO domain and the easy axis, on applied voltage pulse, compared with the polarization of the BFO layer versus applied voltage measured at 9.5 GHz. Error bars in c are defined as the s.d. of five FMR measurements for each FMR data. Error bars in d are deducted by the error of FMR measurements. Full size image The above experimental observations cannot be explained by conventional magnetoelectric coupling mechanisms, such as charge-mediated magnetoelectric coupling [20] , [21] , [22] , [23] , or strain-mediated magnetoelectric coupling [10] , [11] , [12] , [18] , [19] , for the following reasons. The IP anisotropic FMR field dependence on applied voltage along different magnetic field orientations is not likely to originate from interfacial charge-screening effects [20] , [21] , [22] , [23] , even though the BFO layer has a high polarization. Charge-screening effect provides an effective OOP magnetic anisotropy to the magnetic thin film [21] , [22] , [23] , [24] ; therefore, the voltage-induced IP FMR field shift due to charge-screening effect should be isotropic with varying α , which is in contrast to our measurements. The observed anisotropic voltage dependence of the FMR field is also not likely to be dominated by strain-mediated magnetoelectric coupling, as strain-mediated magnetoelectric coupling will be diminished by substrate clamping effects [18] , [19] . Furthermore, it has been previously demonstrated that the coupling between the BFO and CoFe vanishes when a few nm thick, fully strained SrTiO 3 layer is interposed between them [13] . Theoretical analysis of E-field control of CoFe/BFO To understand the voltage-dependent FMR data, we consider a CoFe layer exchange coupled to the canted moments of a BFO layer within the two ferroelectric domains as shown in Fig. 3a [13] , [14] , [15] , [16] , [17] . The canted magnetic moment orientations (green and orange) in the two ferroelectric domains (red and blue, respectively) of the BFO thin film are perpendicular to each other [13] . Within a single BFO unit cell, the polarization ( P ) lies along a <111> direction. The canted moment ( M C ) and the antiferromagnetic axis ( L ) are perpendicular to each other in a (111) plane [13] , [14] , see Fig. 3a and Supplementary Fig. 3 , with L along <1–10> direction and M C along <11–2> direction. Thus, on this (001) surface of the BFO film, the total net IP polarization and the total net IP canted moment in BFO project parallel to each other along the (1–10) DSO direction, which is perpendicular to the stripes as shown in Figs 1c and 3a and Supplementary Fig. 3 [33] . Under an OOP electric field, the polarization in each of the two BFO domains is rotated by 180° as illustrated on the right side of Supplementary Fig. 3 and confirmed experimentally by the PFM images shown in Fig. 3b . Both the IP, ( Fig. 3b , left, black arrows), and OOP, ( Fig. 3b , right), components of the polarization of BFO domains reverse from the as-grown (left side) to the switched state (right side). Therefore, the total polarization of BFO is rotated by 180° under an OOP E-field. These experimental results are confirmed by phase field modelling as shown in Supplementary Fig. 2 , which clearly reveals the two-step switching of the polarization vector under an OOP applied electric field. The measured α angle dependence of the FMR field is shown in Fig. 3c . Within the picture presented in our model, M C and M CoFe are parallel on the blue curve so less FMR field is required to attain the resonance condition. On the red curve, M C and M CoFe are antiparallel so the FMR field must be larger. The FMR field at α =0° and 180° can be switched by a voltage pulse back and forth from the blue curve to the red curve, from 217 to 225 mT, that is, a tunable FMR field range of 8 mT. In contrast, the FMR fields at α =90° and 270°, show nearly no change with voltage pulse. These results are consistent with the experimentally observed FMR field versus applied voltage loops at different α angles shown in Fig. 2c . The difference between the FMR field measured at α =0° and α =90° of 5.1±0.5 mT (the blue curve) and 2.9±0.3 mT (the red curve) from Fig. 3c is the combination of the growth anisotropy field and the net IP magnetic anisotropy field induced by the exchange coupling [13] between CoFe layer and BFO layer. The growth anisotropy field was found to be 1.1±0.2 mT. The net IP exchange coupling field, H EXeff , was determined to be 4±0.3 mT, which is scaled by 1/cos 45° to give H EX =5.7±0.4 mT (see Supplementary Methods , modelling the FMR field and β angle dependence on applied voltage) This value is comparable to a previously reported value for the IP exchange coupling determined by a complementary method [17] . To further our understanding of the coupling, we measure FMR fields as we vary α without switching the voltage, which complements our usual measurements taken by switching voltage pulses at fixed α angle. In particular, after a voltage pulse switched from point 1 to point 4 in Fig. 3c , we maintain the +0 V polarization state and rotate the applied magnetic field direction from 0° to 180°. The FMR field follows the red curve from point 4 to point 3 at α= 90°, but then follows the blue curve to point 2 at α= 180° instead of to point 5. When the applied magnetic field is rotated back from 180 to 0°, the FMR field remains on the blue curve, changing from point 2 to point 3, at α =90°, and back to point 1, instead of to point 4. This measurement demonstrates that the +0-V points (red curve) correspond to a metastable state that is created by applying an electric field pulse, and that this metastable state can be switched to a more stable −0 V ground state (blue curve) by rotating the bias field through α =90° or α =270° where the states are degenerate. This instability explains why a voltage-induced exchange bias is not observed in hysteresis measurements of this system [13] . Finally, to reaffirm the coupling between BFO and CoFe, it is critical to carry out a ‘null’ experiment. We deposited Cu (3 nm)/CoFe (1.2 nm, 2.5 nm) bilayers in a 20-mT in situ magnetic field on a 50-nm SrTiO 3 (STO) dielectric thin film. We measured the FMR signal on the CoFe/STO heterostructure at different voltages across STO following the same procedure as for the CoFe/BFO heterostructures. No FMR field shift was observed in CoFe (2.5 nm)/STO (50 nm) heterostructure, see Supplementary Fig. 4 . The calculations and discussion are listed in the Supplementary Methods , experimental and theoretical study of FMR measurements in a CoFe/STO multiferroic heterostructure ( Supplementary Fig. 4 ). With this compelling experimental data as the framework, we present a model that allows us to understand what happens to the canted moments in each of the BFO domains’ exchange coupled to the CoFe. Unfortunately, little is known about the magnetic structure and energetics of the CoFe/BFO interface so several coupling models may be possible. However, a model must be consistent with our experimental observations: namely, the uniaxial anisotropy, the hysteretic switching of FMR fields, the voltage-induced metastable state and the degenerate nature of the structures at α =90° and α =270°. A model, which describes the data well, is based on the assertion that the IP M C is either parallel or antiparallel to the IP P , and that P reverses with voltage but does not change when the magnetic field is rotated. When P is rotated 180° by an OOP E-field, the voltage-induced system energy change overwhelms the CoFe/BFO canted moment interface exchange coupling energy, creating an energy barrier that allows the canted moment in BFO to be in a metastable state antiparallel to the magnetization direction of CoFe. Although the coupling between M CoFe and M C is unidirectional, it becomes unstable at α =90° and thereby approximates a uniaxial anisotropy (see Supplementary Methods , modelling the FMR field and β angle dependence on applied voltage). To calculate the BFO-canted magnetic moment rotation angle quantitatively from the FMR measurements and to simulate the voltage dependence of the angular variation of the FMR field, we used the coordinate system in Fig. 3a . As discussed in the Supplementary Methods section, the voltage-dependent FMR field of CoFe at different α angles can be quantitatively simulated as shown by the dashed line in Fig. 3c . Also, by substituting the experimentally determined angle-dependent FMR field shift into the energy functional, we can deduce the dependence of β (V) on applied voltage pulse. The hysteretic β (V) versus applied voltage curve (blue) obtained from the model closely matches the P–E polarization hysteresis loop (red) as seen in Fig. 3d . Suppose the two states 0+ and 0− refer to two different remnant polarization states at 0 V where the 0− is initial state. We can solve for the angle β at both 0+ and 0− state as: The analytical results indicate that β (V) in the single domain (red) was switched from ≈45° to ≈−135° with changing applied voltage pulses, which confirms the ≈180° reversal of the canted magnetic moment by the E-field is in agreement with the schematic of Supplementary Fig. 3 . In conclusion, we present angle-dependent FMR field shifts demonstrating a voltage pulse induced, robust, repeatable switching of the magnetic coupling in a CoFe/BFO thin-film heterostructure. The canted moment in BFO does reverse direction with the application of a bipolar electric field. This work demonstrates the significant potential for exchange coupled magnetic film/BFO heterostructures in spintronics devices for compact, fast, energy-efficient voltage-writable RF/microwave and spintronics/MERAM devices. Thin-film fabrication Pt (2.5 nm)/Co 0.9 Fe 0.1 (2.5 nm)/(001) BiFeO 3 (200 nm)/SRO (10 nm) multilayer was grown onto (110)-oriented DSO substrates using pulsed laser deposition. The Pt(2.5 nm)/Co 0.9 Fe 0.1 (2.5 nm) bilayers were deposited under a 20-mT in situ bias magnetic field along the DSO(1–10) direction. Cu (3 nm)/CoFe (1.2 nm, 2.5 nm)/STO (50 nm)/Pt (10 nm) multilayer was deposited by physical vapour deposition on (001)-oriented Si substrate. Circular CoFe disks were obtained by ion milling from full film (10 μm diameter for domain structure imaging, 200 μm diameter for FMR measurements). Characterization The magnetic domain structure of the CoFe layer at zero magnetic field was imaged using scanning electron microscopy with polarization analysis (SEMPA). The ferroelectric domain structure was imaged using PFM. All FMR measurements by electron spin resonance system (X-band, 9.5 GHz) under ~200 mT external magnetic field. Electric field was applied across BFO and STO layer. Micromagnetic simulations of magnetic coupling between BFO and CoFe To understand how the rotation of polarization affects the magnetic moment, micromagnetic simulation was performed for a heterostructure of (CoFe/BFO) [40] . Coupling with the polarization fixes the easy axis of the AFM spins in each BFO domain and spin canting in BFO creates weak ferromagnetism that couples to CoFe. The micromagnetic simulation takes into account the exchange coupling of the CoFe spins and the exchange coupling between the CoFe spins and BFO spins simultaneously. Supplementary Fig. 1a shows the initial condition and Supplementary Fig. 1b shows the configuration after a vertical electric field was applied to the BFO causing it to switch by 180°. It is found that while the CoFe spins follow the configuration of the underneath ferroelectric domains closely, these competing interactions lead to deviation from perfect 90° configuration of the adjacent domains, exactly as observed in the SEMPA data. It is also observed that the domain size changes as it is also found in the experiment. Note that the coupling between the canted moment and CoFe spins indicate that as the CoFe domains get reoriented, the canted moment is also changed from its equilibrium position. Indeed an enhanced moment of 1–2 μB per unit cell was predicted for the case where the exchange bias is small and coercivity is ~5 mT (very similar to the current experiment). Phase field modelling of two-step ferroelectric switching in BFO For a vertical electric field, the polarization switches by 180° in each unit cell as opposed to the case with a lateral electric field [37] where in each unit cell, the polarization switches only by 90° and two adjacent domains together provide a net rotation of polarization by 180°. However, even for the vertical electric field, where the polarization in each unit cell is switching by 180°, the switching goes through a two steps process. Imagine the polarization in the blue region shown in Supplementary Fig. 2 was originally pointing to the bottom left corner in the front. Once an electric field in the up direction is applied, this polarization rotates to the top left corner in the front (see the middle figure). However, this position is not strain compliant with the surrounding of the film due to the fact that the distortion of the unit cell will now be orthogonal to the global distortion in the film. Therefore, an elastic rotation ensues and rotates the polarization to the top right corner in the back. This rotation projects as an 180° rotation on the (001) surface. Thus the projection of the polarization switches by 180° on the (001) surface. How to cite this article: Zhou, Z. et al. Probing electric field control of magnetism using ferromagnetic resonance. Nat. Commun. 6:6082 doi: 10.1038/ncomms7082 (2015).